Continuous wireless pressure monitoring and mapping with ultra-small passive sensors for health monitoring and critical care Continuous monitoring of internal physiological parameters is essential for critical care patients, but currently can only be practically achieved via tethered solutions. Here we report a wireless, real-time pressure monitoring system with passive, flexible, millimetre-scale sensors, scaled down to unprecedented dimensions of 1 × 1 × 0.1 cubic millimeters. This level of dimensional scaling is enabled by novel sensor design and detection schemes, which overcome the operating frequency limits of traditional strategies and exhibit insensitivity to lossy tissue environments. We demonstrate the use of this system to capture human pulse waveforms wirelessly in real time as well as to monitor in vivo intracranial pressure continuously in proof-of-concept mice studies using sensors down to 2.5 × 2.5 × 0.1 cubic millimeters. We further introduce printable wireless sensor arrays and show their use in real-time spatial pressure mapping. Looking forward, this technology has broader applications in continuous wireless monitoring of multiple physiological parameters for biomedical research and patient care. Monitoring physiological variables such as pressure, pH, oxygen level and glucose is essential to routine biomedical research and clinical practice. Patients in critical care units are typically monitored at regular intervals, and often continuously, so that medical staff can track their physiologic status in real time. However, continuous monitoring of these physiological parameters currently requires tethered, wired connections [1] . For example, use of an implanted catheter with an external transducer is standard for monitoring intracranial pressure (ICP) in patients suffering from head trauma [2] . The ability to assess intracranial hypertension continuously is the key to prompt intervention and favourable outcomes. However, tethered solutions cause patient discomfort and carry a risk of infection, and complications stemming from dislodgement, leakage and blockage. Early attempts at passive (non-tethered) solutions operated at low frequencies, which require relatively large components and translate to sensor size in the cm 3 range [3] , [4] , [5] , [6] , [7] , [8] , [9] , [10] . Although their development has ceased, emerging wireless solutions specifically for ICP monitoring have also had large sizes, as they use batteries and active circuitry to power the sensor device [11] , [12] , [13] , [14] , [15] , [16] , [17] , [18] . The smallest wireless pressure monitoring device to date is a battery-powered wireless sensor that researchers have fit into a 1-mm 3 package for intraocular applications [19] . Several groups have been able to successfully reduce the integrated circuit (IC) chip size down to 2.5–4.5 mm 2 for actively powered wireless pressure devices, but they still require a separate 5–6 mm diameter antenna coil [20] , [21] . Recently, microfabrication techniques and microelectromechanical system technology have been applied to reduce device footprints in passive wireless sensing of intraocular pressures [18] , [19] , [20] , [21] , [22] . However, with all the sensors operating below a few hundred MHz, none has been able to miniaturize below a few mm 3 in volume [3] , [4] , [5] , [6] , [7] , [8] , [9] , [10] , [22] , [23] , [24] , [25] , [26] . Traditional passive strategies have been inherently limited by the self-resonant frequency of readout circuitry because interference effects make it difficult to detect sensors operating near and above this frequency [27] , [28] , [29] . There is a significant need to miniaturize monitoring devices to make them less traumatic and easier to implant. We introduce a scalable system of passive, millimetre-scale sensors, plus a wireless detection scheme designed to overcome the operating frequency limits of traditional passive strategies. Mechanical flexibility is expected to give the device improved mechanical robustness over brittle devices, and would allow the sensor to be used on non-planar surfaces after calibrating for bending-induced changes in sensor characteristics. We present the design and characterization of this continuous pressure monitoring system with wireless devices in the following sections. We first describe a size scaling path to achieve the smallest passive sensors reported for wireless pressure monitoring, with dimensions of 1 × 1 × 0.1 mm 3 . At a volume of 0.1 mm 3 , this is more than an order of magnitude smaller than previously reported research devices [22] , [23] , [24] , [25] , [26] and more than two orders smaller than commercial solutions [15] , [16] , [17] , [18] . We apply this system to capturing human radial pulse waveforms in real-time with externally placed wireless sensors. We further present proof-of-concept studies of real-time in vivo ICP monitoring in mice with sensors down to 2.5 × 2.5 × 0.1 mm 3 . Concurrent spatial pressure mapping is demonstrated with printable wireless sensor arrays. Passive resonant sensors We integrate a pressure-sensitive capacitive element with an inductive antenna to form a resonant circuit, which has a unique resonant frequency under zero pressure. To achieve size scalability, we create a distributed resonant tank by stacking a deformable dielectric layer between the two inductive spirals in a sandwich structure, as shown in Fig. 1a . Under applied pressure, the separation distance between the spiral layers is reduced, increasing the effective coupling capacitance and shifting the resonant frequency down to lower frequencies. The spiral layers are printed or lithographically patterned on flexible polyimide substrates, while the pressure-sensitive dielectric layer is implemented with a microstructured styrene-butadiene-styrene (SBS) elastomer. The microstructured elastomer and final assembled sensor are shown in Fig. 1b,c , respectively. Scanning electron microscopy images of the electrodes and patterned dielectric layer are included in Supplementary Fig. 1 . The microstructured elastomer dielectric has previously been shown to be more sensitive than its unstructured counterpart [30] . The improved sensitivity is due to reduced viscoelastic behaviour of thin films and the change in effective permittivity of the region between the plates under compression, in addition to the change in separation distance. The pyramidal elastomer microstructures deform to fill in the air gaps between them with applied pressure, thus increasing the effective permittivity. This sandwich form enables a simple low-cost method of wax printing process by eliminating the need for vias to connect discrete inductive and capacitive structures in parallel. We used SBS instead of other commonly known elastomers, such as poly(dimethyl siloxane) (PDMS) or polyurethane, due its low loss in the high frequency range [31] . However, one drawback when using SBS is the drift in capacitance values during cycling measurements, as seen in Supplementary Fig. 2 . 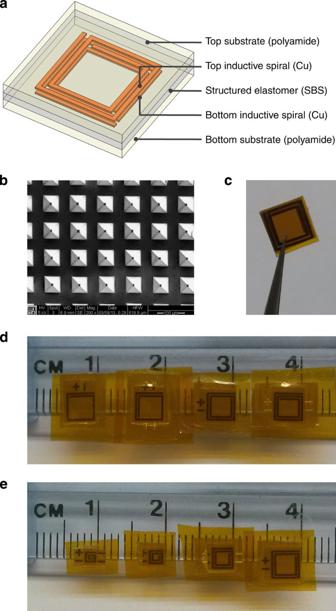Figure 1: A 4 × 4 mm22-turn resonant sensor device. (a) Structure design. (b) Optical image of pyramidal structured SBS dielectric. (c) Photograph of assembled device. Assembled (d) 4 × 4 mm2devices with 1.25, 1.5, 2 and 2.25 turns and (e) 2-turn devices scaled from 4 × 4 mm2to 1.5 × 1.5 mm2. Figure 1: A 4 × 4 mm 2 2-turn resonant sensor device. ( a ) Structure design. ( b ) Optical image of pyramidal structured SBS dielectric. ( c ) Photograph of assembled device. Assembled ( d ) 4 × 4 mm 2 devices with 1.25, 1.5, 2 and 2.25 turns and ( e ) 2-turn devices scaled from 4 × 4 mm 2 to 1.5 × 1.5 mm 2 . Full size image Wireless detection Wireless operation is achieved through near-field electromagnetic coupling between the resonant sensor device and an external antenna. This external antenna is connected to the continuous wave (CW) readout system, as illustrated in Supplementary Fig. 3 . We leverage the variable frequency CW source generation, incident and reflected wave isolation capabilities of a vector network analyser (VNA) to implement the readout system. The VNA is controlled directly by a Matlab programme and connected to the readout antenna through a flexible cable as shown in Supplementary Fig. 4a,b . The readout system can be programmed to detect and characterize sensors by searching for the peak power reflection change over the captured input frequency spectrum. We can define a power reflection distortion (PRD) quantity below as the function of input reflection coefficients Γ in with and without a resonant sensor present, The input reflection is minimal near the sensor resonant frequency when power is maximally absorbed by a resonating sensor. Through theoretical analysis of an RLC sensor circuit inductively coupled to a readout coil, it is shown that this maximum in the PRD spectrum occurs close to the sensor resonant frequency within a small error that varies inversely with the square of the sensor quality factor Q senor , Power absorption is media dependent and is sensitive to lossy environments such as human tissue. To mitigate such effects, we introduce another CW method to identify sensor resonance at the external readout antenna by searching for the greatest change in reflection group delay with a software maximum function. The reflection group delay is found by differentiating the phase response of a system with respect to frequency. We define a group delay distortion (GDD) quantity to be the following function of the complex-valued input reflection coefficients Γ in with and without a resonant sensor present, Analysis shows the difference in group delay becomes maximal near the sensor resonant frequency within a small error that again varies with the inverse square of the sensor quality factor, In practice, the readout system is also first calibrated to determine the reference spectrum in the absence of the sensor as well as a baseline noise level. To detect the sensor resonance, we trigger excitation from the VNA over a linear sweep over a fixed frequency range and capture a resultant input reflection spectrum. An averaged sequence of these reflection spectrum is taken and a median filter is applied to remove white noise. The measured input reflection spectrum is squared in software and subtracted by the square of the reference spectrum to generate the PRD spectrum. The GDD spectrum is similarly derived from the first derivative of measured input reflection and reference spectrum in software. In continuous monitoring, we run the resonant peak detection in a loop while rejecting peaks, which fail to meet a signal-to-noise ratio threshold of 3 dB. In array monitoring, multiple peaks are distinguished by dividing up the spectrum into frequency bands based on a signal-to-noise threshold. Device and system characterization The resonant frequency and spatial range over which a sensor can be detected are characterized for a fixed device area (4 × 4 mm 2 , Fig. 1d ) with varying number of turns, and also for a fixed number of turns (2-turn) with device area scaled from 4 × 4 mm 2 down to 1.5 × 1.5 mm 2 ( Fig. 1e ). The plot of resonant frequencies for devices of varying spiral lengths in Fig. 2a shows that increasing spiral length reduces device resonant frequency. The measured values in Fig. 2a are in good agreement with analytical model and simulated predictions. As either device area or number of turns is scaled down, the sensor resonant frequencies increase and the sensor begins to operate in a regime near and above the self-resonance of the readout antenna. For instance, a 4 × 4 mm 2 readout antenna is inductive at low frequencies but exhibits self-resonance near 2 GHz. This self-resonance causes a magnitude peak and phase reversal in the input impedance measured at the readout antenna but produces no discernible disturbance in the PRD and GDD spectra. Hence, sensor resonant peaks can be distinguished with the PRD and GDD detection schemes even at high frequencies, independent of the readout antenna design. 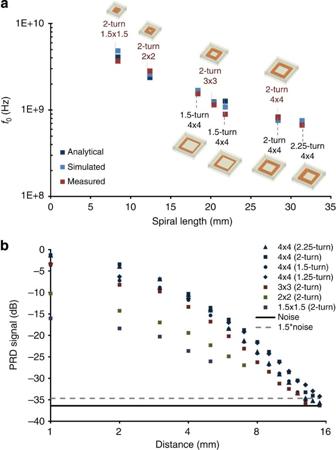Figure 2: Design variations and their performance. (a) Analytical, simulated and measured resonant frequency versus spiral length for 4 × 4 mm2devices with varying turns and 2-turn devices scaled from 4 × 4 mm2to 1.5 × 1.5 mm2. (b) Measured PRD peak signal degradation with spatial distance between readout antenna and sensor device for 4 × 4 mm2devices with varying turns and 2-turn devices scaled from 4 × 4 mm2to 1.5 × 1.5 mm2. Figure 2: Design variations and their performance. ( a ) Analytical, simulated and measured resonant frequency versus spiral length for 4 × 4 mm 2 devices with varying turns and 2-turn devices scaled from 4 × 4 mm 2 to 1.5 × 1.5 mm 2 . ( b ) Measured PRD peak signal degradation with spatial distance between readout antenna and sensor device for 4 × 4 mm 2 devices with varying turns and 2-turn devices scaled from 4 × 4 mm 2 to 1.5 × 1.5 mm 2 . Full size image The maximum spatial distance from which the sensor can be detected is determined by the point at which the peak PRD or GDD magnitude falls below the minimum distinguishable signal level. Figure 2b shows PRD peak signal degradation with increasing distance between the readout antenna and the sensor device. We are able to achieve up to 15 mm in spatial range with the 4 × 4 mm 2 device in an air environment. Scaling down sensor dimensions shifts the curve down to lower signal levels in accordance with scaling of the effective aperture size of the resonant sensor antenna. For the same device dimensions, relatively small differences in the spiral length do not considerably have an impact on the sensor range ( Fig. 2b ). To test the wireless sensor response over a broad range of pressures, we used a gas pressure chamber to apply different pressures ( Supplementary Fig. 4b ) relative to atmospheric pressure. The resonant peak in the PRD and GDD spectra shifts down in frequency in response to applied pressure as shown for a 2-turn 4 × 4 mm 2 device in Fig. 3a,b , respectively. Sweeping over a pressure range of 500 mm Hg generates the pressure calibration curve in Fig. 3c . The pressure response is very linear in the physiologic pressure region of 0–100 mm Hg, with a Pearson correlation coefficient of 0.99. The sensor exhibits reduced sensitivity at pressures beyond 100 mm Hg. This behaviour is similar to the capacitive pressure sensor-based microstructured rubber we previously reported, and the origin was also previously discussed [28] . 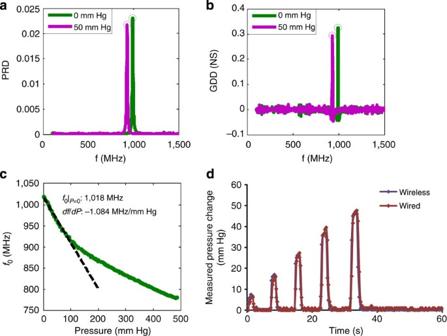Figure 3: Pressure response of a 2-turn 4 × 4 mm2sensor device. Shift in the resonant peak in the measured (a) PRD and (b) GDD spectra. (c) Sensor resonant frequency change with applied pressure over 500 mm Hg range. (d) Real-time pressure response as measured by wireless sensor device and reference wired sensor during continuous monitoring. Pressure values are reported relative to atmospheric pressure. In the linear region, we can use the simple expression below to translate peak frequency measurements f 0 into physical pressure values P ( f 0 ), Figure 3: Pressure response of a 2-turn 4 × 4 mm 2 sensor device. Shift in the resonant peak in the measured ( a ) PRD and ( b ) GDD spectra. ( c ) Sensor resonant frequency change with applied pressure over 500 mm Hg range. ( d ) Real-time pressure response as measured by wireless sensor device and reference wired sensor during continuous monitoring. Pressure values are reported relative to atmospheric pressure. Full size image The zero pressure intercept f 0 | P =0 and pressure sensitivity are derived from a linear regression of the pressure calibration curve over the 0–100 mm Hg region. Using this measured calibration curve with PRD detection of the sensor resonant frequency, we continuously monitor the same 2-turn 4 × 4 mm 2 device over a 1-min period. The real-time pressure waveform captured wirelessly in Fig. 3d tracks well with that measured with a wired reference sensor having the same device structure and feature size in the gas chamber pressure controller. A similar wired device was used to characterize the bending dependence of the capacitance change ( Supplementary Fig. 5 ). We found that bending of the sensor will indeed affect the output signal. However, this issue can be partially addressed by using thinner substrates. In addition, many applications do not require change of bending radius during measurements. For example, in the ICP measurement to be discussed below, the sensor is fixed at a certain bending radius. After the initial bending during device placement, there is no further change in bending radius subsequently. In preparation for in vivo studies, we characterize a 2-turn 3 × 3 mm 2 sensor device in saline. We have chosen a smaller size for ease of implantation in small animals. The lossy nature of human tissue is modelled with a saline phantom by modifying the gas chamber setup for fluid environments ( Supplementary Fig. 4c ). 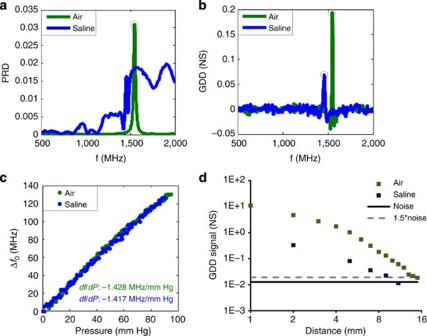Figure 4: Characterization of a 2-turn 3 × 3 mm2implant sensor in saline. Measured (a) PRD and (b) GDD spectrums of implant sensor under no applied pressure in air and in saline. (c) Sensor resonant frequency change with applied pressure over 500 mm Hg range in air and in saline. Pressure values are reported relative to atmospheric pressure. (d) Measured GDD peak signal degradation with spatial distance between readout antenna and sensor device in air and in saline. Figure 4a shows that the resonant peak in the PRD spectrum becomes masked due to baseline interference. On the other hand, as shown in Fig. 4b , the GDD spectrum baseline is largely unaffected, while the resonant peak decreases in magnitude and shifts to lower frequency. As these studies have revealed the weakness of PRD scheme in saline environments, we opted to operate our system with GDD scheme in all subsequent studies. The drift observed is due to slow diffusion of water through the polyimide substrate and the adhesive. We can potentially subtract this shift after carefully characterizing the shift over time and build this into our data analysis. We can also replace polyimide with other substrates that have lower water permeability or use encapsulation films to reduce water permeation. We find that pressure sensitivity measured in air and saline environments are comparable in Fig. 4c . Figure 4d shows consistently lower peak signal levels in the lossy saline environment than in air at fixed distances between the sensor device and readout antenna. This results in a reduction of the operating distance range to about half that in air. Figure 4: Characterization of a 2-turn 3 × 3 mm 2 implant sensor in saline. Measured ( a ) PRD and ( b ) GDD spectrums of implant sensor under no applied pressure in air and in saline. ( c ) Sensor resonant frequency change with applied pressure over 500 mm Hg range in air and in saline. Pressure values are reported relative to atmospheric pressure. ( d ) Measured GDD peak signal degradation with spatial distance between readout antenna and sensor device in air and in saline. Full size image Smallest wireless pressure sensor Using optical lithography with a minimum feature size and pitch of 25 μm, the sensor size is reduced to 1 × 1 mm 2 with the 5-turn designs. 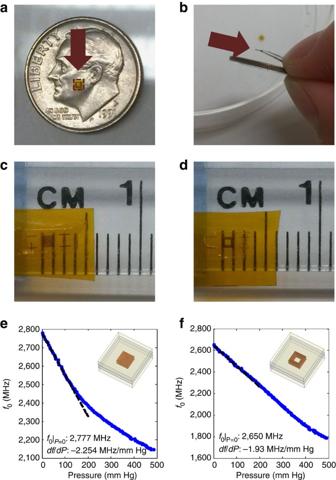Figure 5: Smallest 0.1 mm3sensors. Photographs of an assembled 5-turn 1 × 1 × 0.1 mm3sensor device next to an American dime showing comparative (a) planar size and (b) thickness. Photographs of sensors with (c) 50 and (d) 25 μm wide line traces and spacing, shown next a metric ruler. Sensor resonant frequency change with applied pressure over 500 mm Hg range for sensors with (e) 50 and (f) 25 μm wide line traces and spacing. With a thickness of 0.1 mm, these are the smallest wireless pressure sensor to be reported in the literature—a volume of 0.1 mm 3 (shown next to an American dime, Fig 5a,b ). Further reduction of size is still possible with state-of-art lithography. We selected 25 μm as the feature size used here, as it can be achieved by printing techniques, such as inkjet and gravure printing. At present, these sensors can be detected within 3 mm. A 5-turn design with wider 50 μm metal traces and spacing in Fig. 5c has the highest sensitivity of 2,254 kHz per mm Hg in its low-pressure linear region of 0–100 mm Hg, as shown in Fig. 5e . A more compact design in Fig. 5d with thinner 25 μm line widths and closer 25 μm spacing has lower sensitivity but is linear over a wider pressure range up to 400 mm Hg, as shown in Fig 5f . The former design covers a larger effective capacitive plate area allowing for greater enhancement effect of permittivity and thus achieving higher sensitivity at low pressures. On the other hand, the latter is linear over a greater range of pressures because the permittivity enhancement at low pressures is negligible with fewer microstructures between the smaller effective capacitor plates. Figure 5: Smallest 0.1 mm 3 sensors. Photographs of an assembled 5-turn 1 × 1 × 0.1 mm 3 sensor device next to an American dime showing comparative ( a ) planar size and ( b ) thickness. Photographs of sensors with ( c ) 50 and ( d ) 25 μm wide line traces and spacing, shown next a metric ruler. Sensor resonant frequency change with applied pressure over 500 mm Hg range for sensors with ( e ) 50 and ( f ) 25 μm wide line traces and spacing. Full size image Pulse waveform monitoring We demonstrate the ability of this system to track human arterial pulse waveform with wireless sensors. A modified round 2.5 × 2.5 mm 2 sensor device was placed on the radial artery of a healthy adult male subject and secured with silicone tape as shown in Fig. 6a . The readout antenna was placed directly above the wireless surface sensor. The pressure waveform was wirelessly measured with the readout antenna in real time. 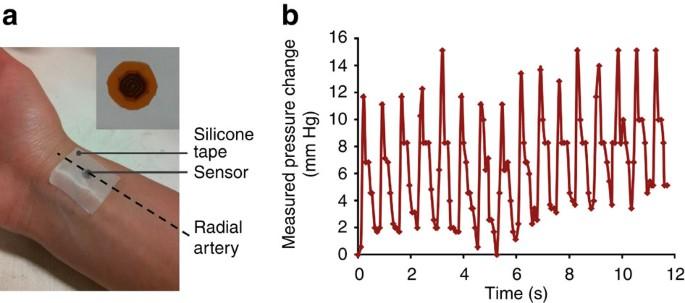Figure 6: Wireless radial pulse monitoring. (a) Placement of a modified 2.5 × 2.5 mm2round sensor shown in inset on the radial artery of a human subject. (b) Measured pulse pressure waveform of a human subject with a heart rate of 82 b.p.m. over 12-s period with a time resolution of 90 ms. Figure 6b gives a sample pressure tracing, which is captured over a period of 12 s with a 0.3-mm Hg pressure resolution and a 90-ms time resolution. The measured waveform possesses the typical profile of an arterial pulse waveform and clearly indicates a steady pulse of about 82 b.p.m. We note that the characteristic pulse waveform shape can be obtained—the peak systolic wave followed by the dicrotic notch, the latter related to the aortic valve closure [32] . Compared with pulse waveform measurement using wired devices, a small wireless device could impose fewer constraints on body movements, and the sensor signal could be perturbed less by such movements. Figure 6: Wireless radial pulse monitoring. ( a ) Placement of a modified 2.5 × 2.5 mm 2 round sensor shown in inset on the radial artery of a human subject. ( b ) Measured pulse pressure waveform of a human subject with a heart rate of 82 b.p.m. over 12-s period with a time resolution of 90 ms. Full size image In vivo validation We studied sensor performance when implanted in mice to further validate this system in vivo . In separate mouse experiments ( N =3), we implanted two 3 × 3 mm 2 sensors and one modified round 2.5 × 2.5 mm 2 sensor in the epidural space through 4 × 5 mm 2 openings in the skull. After the scalp was closed with sutures, an external antenna was placed directly outside the implantation site, as shown in Fig. 7a,b , which demonstrates clear detection of the sensor resonance peak in the GDD spectrum of the external readout antenna. The shift in zero pressure resonant frequency is due to higher dielectric permittivity of the mouse tissue environment and it is comparable to that predicted by characterization in saline. 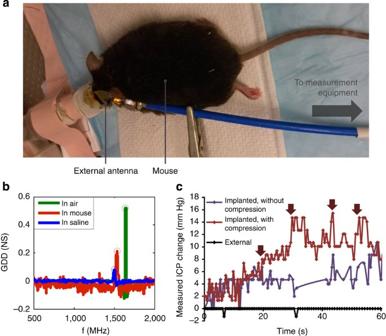Figure 7: Wireless ICP monitoring with the 2-turn 3 × 3 mm2sensor implanted in mouse. (a) Placement of external antenna. (b) Detected sensor resonant peak in the measured GDD spectrum under no applied pressure in air, in saline and in mouse. (c) Pressure waveforms as measured over 60-s period with an implanted 3 × 3 mm22-turn sensor with and without performing abdominal compression on mouse and with an external reference sensor. The arrows correspond to when compression was applied. Figure 7: Wireless ICP monitoring with the 2-turn 3 × 3 mm 2 sensor implanted in mouse. ( a ) Placement of external antenna. ( b ) Detected sensor resonant peak in the measured GDD spectrum under no applied pressure in air, in saline and in mouse. ( c ) Pressure waveforms as measured over 60-s period with an implanted 3 × 3 mm 2 2-turn sensor with and without performing abdominal compression on mouse and with an external reference sensor. The arrows correspond to when compression was applied. Full size image We continuously tracked pressure changes from an initial zero pressure frequency measured immediately following implantation. Abdominal compressions were performed to forcibly induce increases in ICP. As compared with an external device under no applied pressure, a baseline pressure drift is observed in Fig. 7c for implanted devices in the absence of abdominal compressions. Induced pressure increases under abdominal compressions are confirmed in the measured waveform above the baseline drift. Pressure mapping As a demonstration of pressure mapping capability, we fabricated a flexible 2 × 2 array of four 2 × 2 mm 2 sensors. Each pressure sensor in the array is designed with a unique resonant frequency from which it can be individually addressed. A sensor’s nominal zero-pressure resonant frequency can be tuned by systematically varying the spiral length as illustrated in Fig. 8a . We chose to space adjacent sensors at least one sensor dimension apart to minimize cross-coupling. The sensor array was fabricated by first etching copper films on flexible polyimide sheets using printed wax as an etch mask (see Methods). The elastomer microstructures are then moulded onto the patterned copper films. 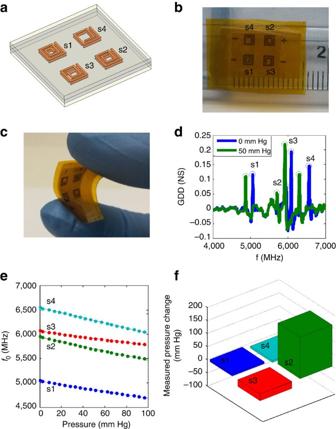Figure 8: Pressure mapping with 2 × 2 flexible array of 2 × 2 mm2sensors. (a) Structure design of 2 × 2 array with sensors labelled s1 through s4. Photographs of sensor array showing (b) size next a metric ruler (c) flexibility when bent. (d) Shift in distinct resonant peaks of all four sensors in the measured GDD spectrum under applied pressure. (e) Simultaneously tracked resonant frequency change with applied pressure of all sensors in the array over 100 mm Hg range. (f) Snapshot of measured pressure map under differential pressure applied on sensor s2. Figure 8b,c show the assembled sensor array in its flat and bent forms, respectively. The resonant peaks of all four sensors in the array can be detected in Fig. 8d at a distance of 5 mm from a single readout antenna in an air environment. The increasing resonant frequency of sensors s1 to s4 validates the presented design methodology. Applying uniform pressure to the sensory array shifts all resonant peaks down in frequency. Individual pressure sensitivity can be quantified by tracking all sensors simultaneously while sweeping the uniform applied pressure. A single calibration sweep produces all four distinct calibration curves in Fig. 8e . Finally, we apply a differential pressure to sensor s2 and characterize individual sensor resonant frequency shifts. The pressure map measured before and after the differential pressure application on the array in Fig. 4f confirms pressure concentration on sensor s2. Figure 8: Pressure mapping with 2 × 2 flexible array of 2 × 2 mm 2 sensors. ( a ) Structure design of 2 × 2 array with sensors labelled s1 through s4. Photographs of sensor array showing ( b ) size next a metric ruler ( c ) flexibility when bent. ( d ) Shift in distinct resonant peaks of all four sensors in the measured GDD spectrum under applied pressure. ( e ) Simultaneously tracked resonant frequency change with applied pressure of all sensors in the array over 100 mm Hg range. ( f ) Snapshot of measured pressure map under differential pressure applied on sensor s2. Full size image In this work, a wireless real-time monitoring system has been demonstrated with passive, flexible millimetre-scale sensors as small as 1 × 1 × 0.1 mm 3 . These devices are more than an order of magnitude smaller in volume than recent research devices for intraocular pressure sensing [22] , [23] , [24] , [25] , [26] and more than two orders smaller than commercial solutions [15] , [16] , [17] , [18] . We are able to achieve this level of scaling by leveraging the presented GDD detection scheme, which overcomes the operating frequency limits of traditional strategies and exhibits insensitivity to lossy tissue environments. This system is used to capture human pulse waveforms in real time as well as to continuously monitor in vivo ICPs with sensors down to 2.5 × 2.5 × 0.1 mm 3 in proof-of-concept mice studies. Furthermore, printable wireless sensor arrays are introduced and their use in concurrent spatial pressure mapping is shown. Even though previous work have converted measurements to frequency changes, the novelty of this work lies in the pressure sensor design that allowed ultra-thin and ultra-small flexible sensors, as well as the readout scheme. The proposed sensor design and detection scheme allow for a highly size-scalable system of pressure sensors with a wireless detection platform. Systematic design and tuning of these sensors by inductive spiral length is enabled with an analytical model, which is shown to agree with simulated and measured results. The greatest deviation between analytical calculations, electromagnetic simulations and measured resonant frequencies is observed with the smallest sensor. This is probably due to an overestimation of inductances at high spiral fill ratio by analytical models [33] . Effective spiral length is desirable for improved mutual coupling to the readout antenna in the near field. This relationship is analogous to that of the number of inductor turns to mutual inductance in a transformer. However, the benefit of increasing effective spiral length is diminishing as thinner and more tightly spaced spirals are fit into a given area because parasitic resistances and capacitances become considerable. The 0.1-mm 3 device is designed with five turns, which is the maximum achievable in a 1-mm 2 area with a minimum feature size and pitch of 25 μm. The square design is later modified to remove edges and create a more rounded form factor for comfort and ease of implantation in human pulse waveform and in vivo mouse ICP studies. As we scale down sensor sizes, the minimum resonant frequency achievable with passive structures for a given area increases. In the millimetre range, minimum achievable sensor resonant frequencies are pushed to GHz range. With a readout antenna in the millimetre to centimetre range for sufficient coupling, the sensor resonant frequency will be on the order of or above the readout antenna self-resonance. In contrast, traditional methods in passive sensing can only be operated at low frequencies, below the self-resonance of the readout coil. These techniques rely on detecting the maxima in the real part or the magnitude [3] , [4] , [5] , [6] , [7] , [8] , [9] , [10] , [22] , [23] , [34] of the input impedance or the phase minimum [24] , [25] , [26] , [35] , [36] . Most operate in the MHz range as a result. The readout self-resonance produces a strong peak in the input impedance real and magnitude spectra and phase reversal in its phase spectrum, making detection of nearby sensor resonances difficult. The proposed PRD and GDD detection schemes overcome the low operating frequency limits of current passive strategies. Although we are still bounded by the fundamental tradeoff between the size of a wireless device and the spatial range over which it is detectable, we are able to operate with 4 × 4 mm 2 sensors over a distance of 15 mm in air from the readout antenna, while the smallest 1 × 1 mm 2 sensors operate over about 3 mm. The spatial range of these passive wireless devices cannot compete with that achievable by active methods, making this technology less suitable currently for applications in deep-seated tissues and organs. However, further improvement of device design and materials can potentially increase the spatial range. The use of a microstructured elastomer as the dielectric layer enhances pressure sensitivity in the low pressure range due to an increase in effective permittivity on top of the reduction in separation distance between the spiral layers under compression. The 5-turn 1 × 1 mm 2 design with 50 μm metal traces and spacing outperforms the most sensitive passive wireless pressure previously reported [33] . At pressures above 100 mm Hg, the microstructures are fully deformed and, hence, only the separation distance reductions act to increase the variable capacitance under applied pressure, resulting in a lower sensitivity. High Pearson correlation coefficient of 0.99 for the relationship between applied pressure and measured sensor resonant frequency indicates excellent linearity within the 0–100 mm Hg range. This is sufficient for the purposes of critical care and health monitoring, as physiological pressures fall within this range. The readout system is not very portable in its current form because it is realized with a VNA. As a multi-purpose measurement equipment, the VNA offers functionality over a wide bandwidth beyond the needs of many applications. In future board-level implementations, one can miniaturize the readout system by achieving the swept CW excitation and reflection spectrum acquisition over a limited bandwidth with conventional radio-frequency wireless transceiver architectures. The detection algorithms can be also realized in hardware with a microprocessor. We recognize that the current wireless sensor design may suffer from interference from metal objects and other electronics when such objects are positioned directly between the sensor and detector antennas in inductive coupling. Given the short spatial ranges we are working in, we do not anticipate any significant metal objects will be wedged within the limited region in which local electromagnetic fields could be sufficiently distorted. To achieve the ultra-small, ultra-thin form factor of the implantable/wearable sensor, we envision that the external antenna would be positioned directly outside and near the sensor. We have reported the smallest passive sensors for wireless pressure monitoring at a volume of 0.1 mm 3 . The current state of art in active wireless sensing is a battery-powered intraocular pressure monitor that researchers have been able to integrate into 1 mm 3 volume [19] . They were able to achieve this compact form by vertically assembling two IC chips, a solar cell, battery and microelectromechanical system capacitive sensor. This prototype has been shown to capture pressures every 15 min with a pressure resolution of 0.5 mm Hg in bench top testing, through 5 mm of saline. The device memory can store pressure measurements up to 3 days before requiring an external wireless download. The device battery has a 28-day lifetime without recharging by the integrated solar cell. Solar power harvesting is not practical in most other in vivo applications because the skin is rather optically opaque. Nevertheless, it is important to note that emerging IC fabrication and packaging techniques can help further reduce the size of wireless sensing devices powered by batteries and active circuitry. We have demonstrated continuous monitoring of human radial pulse waveforms in real time with wireless sensors placed superficially on the radial artery. There is a tradeoff between time resolution and measurement resolution in this system. Reducing the number of swept frequency points lowers both computation time and data transfer delays at the expense of precision in measured resonant frequency over a fixed frequency range. Averaging and filtering steps are minor knobs that can be eliminated in continuous monitoring to improve time resolution at the cost of frequency accuracy. For a single measurement, the present implementation takes about 210 ms to acquire 10 sweeps of 1,601 frequency points and read into memory in software. Processing the measured spectra with averaging and filtering in software only takes about 10 ms. This proof-of-concept implementation with a software-controlled network analyser is capable of capturing pressure waveforms with time resolutions down to 20 ms with at least 1 mm Hg pressure resolution by using only 101-point sweeps. The pressure resolution can alternatively be pushed down to below 0.1 mm Hg pressure resolution with the same 20 ms time resolution by limiting the swept frequency range to cover only a 100-mm Hg pressure range. We currently recalibrate the zero-pressure intercept with a known zero-pressure condition directly before the timed measurement to account for any resonant frequency shifts due to changes in the effective permittivity of the deformable dielectric layer and separation of the substrate layers. Causes of such changes include material degradation over time and permanent deformation from excess mechanical stresses. In vivo testing with this system is demonstrated for real-time ICP monitoring in mice. We have implanted and wirelessly detected sensors as small as 2.5 × 2.5 × 0.1 mm 3 with an external readout antenna. The zero-pressure resonant frequency in mouse is similar to that characterized in saline. The shift to lower resonant frequencies and reduction in the effective sensor quality factor is expected due to the higher dielectric constant and loss tangent of tissue and saline as compared with air environments. Sensor resonant frequency can be detected in saline and tissue from the GDD spectrum. Traditional input impedance-based techniques as well as the PRD scheme fail due to considerable interference from the lossy media, particularly at higher frequencies. Electromagnetic field attenuation in the lossy saline medium diminished peak signal levels, thereby cutting down the detectable spatial range. Despite the signal attenuation, we were still able to wirelessly monitor an internal sensor implanted beneath the mouse skull. We observe a gradual decrease of the sensor resonant frequency and, thereby, an upward drift in the measured pressure. This drift is probably due to moisture leaking into the sensor from the mouse tissue environment. The higher permittivity of water causes an increase in the effective permittivity between substrate layers which in turn causes capacitance to increase and sensor resonant frequency to lower. Better encapsulation methods can be applied to reduce this effect, such as replacing the substrates with less permeable materials. Furthermore, this period of instability was avoided by pre-conditioning the sensor in saline before implantation in later experiments. Abdominal compressions performed on mouse with an implanted sensor device are corroborated by pressure elevations in the wirelessly captured waveform on top of a baseline drift. We have shown the additional application of flexible sensor arrays to perform wireless spatial pressure mapping. ICP mapping would be useful in assessing local pressure buildups. Moreover, multiple pressure sensors would allow flow rates to be determined from measured pressure differentials. Determining flow rate is important for cerebrospinal fluid shunt applications in patients with hydrocephalus [2] . Here, the flow rate can be used in a feedback loop to control the shunt valve opening and closing. Each 2 × 2 mm 2 pressure sensor in the prototype planar array is tuned with our analytical models to possess an individually addressable resonant frequency band spaced 350 MHz apart. For a typical pressure sensor with 1 MHz per mm Hg sensitivity, each sensor only needs to occupy a bandwidth of 100 MHz to cover the physiological pressure range of 0–100 mm Hg. This allows all sensors to be concurrently monitored with a single readout antenna. Unique resonant peaks corresponding to individual sensors in the array can be best distinguished in the GDD spectrum. Resonant peaks in the GDD spectrum are sharper than in the PRD spectrum for a sensor of the same quality factor, resulting in less overlap between frequency adjacent sensors. Non-uniform spacing of resonant frequencies and inconsistent pressure sensitivity of the fabricated sensor array can be primarily attributed to process variation. Differential pressure application on sensor s2 has been verified by the measured pressure map. We also observe apparent negative pressure on adjacent sensors s3 and s4. This can be attributed to the lifting of the adjacent sheet corners when the s2 corner is depressed. To achieve independent mechanical deformation of sensors, the single sheet form factor of array needs to be adjusted. Detection of multiple pressure sensors using a single readout antenna is not limited to two-dimensional planar arrays. Sensors can be placed at varying depths arranged in order of increasing Q with increasing depth to ensure the farthest can still be read. In conclusion, we report a wireless sensing system that allows for wireless pressure sensors to scale down to sizes smaller than previously reported in the literature for wireless pressure monitoring. PRD and GDD detection schemes have been introduced that overcome the low frequency barriers of traditional passive methods. We additionally show the insensitivity of the GDD spectrum to lossy media such as saline and tissue, making it a promising candidate for in vivo sensing. The application of this system in real-time external pulse waveform tracking and in vivo ICP monitoring has been shown. We further demonstrate its potential use in pressure mapping through flexible sensor arrays. We anticipate that this technology will open up exciting opportunities in continuous wireless monitoring of other physiological parameters in biomedical research and clinical practice. Design and simulation The sensor device structures are designed, modelled and simulated in Ansoft High Frequency Structure Simulator (HFSS). The electromagnetic coupling between a readout antenna and a resonant device is simulated in HFSS and exported as two-port S parameter model. Full system modelling is achieved by co-simulation of the detection circuit in the RF/microwave circuit simulator Agilent Advanced Design System with a coupled readout and sensor subsystem as 2-port black box network defined by imported HFSS S parameters. PRD and GDD spectrums are derived by also simulating in the absence of sensor. Analytical model The resonant structure in Supplementary Fig. 6 can be analytically modelled to first order with a simple RLC circuit with a resonant frequency f sensor and equivalent angular frequency ω sensor given by Here, the effective inductance L eff can be calculated for an n -turn square spiral with outer diameter d out and inner diameter d in with the modified Wheeler’s formula [24] given below The effective capacitance C eff is computed with a modified parallel plate capacitor formula below in which the effective plate cross-sectional area A eff is the planar surface area of each spiral metal trace and d sep is the separation distance between the spiral layers. A weighted ratio for the permittivity of air ε 0 and of elastomer ε elastomer based on the volume proportion of air V air and of elastomer V elastomer between the parallel plate structure is used. Fabrication Sensors are made in one of two ways: one using a low-cost method of wax printing and the other using standard lithography techniques. In the low-cost method, we used copper coating on top of a flexible polyimide film as substrate. Next, we print a layer of wax pattern onto the copper surface using a commercial wax printer (Xerox Phaser) followed by etching in ferric chloride solution at 50 °C for about 5 min until the non-waxed surface (exposed copper surface) was completely etched away. The wax layer was then removed by sonicating in acetone. In the standard lithography method, we first pattern a layer of photoresist onto a polyimide-coated silicon wafer, followed by thermal evaporation of 900 nm of copper and lift-off of the photoresist layer in acetone. To obtain the elastomer microstructures, we used the previously published technique using soft lithography [30] . We then replicated the silicon mould indentations on PDMS (Sylgard 184, Dow Corning) by performing the mould-making procedure twice, first on the silicon, then on the replicated structures in PDMS, to create a soft lithographic mould identical to the silicon indentations. Next, we mould the thermoplastic elastomer SBS (D1102 from Kraton) as the elastomeric microstructures by spin-coating from a tetrahydrofuran solution with a concentration of 75 mg ml −1 at a speed of 2,000 r.p.m. for 1 min. System implementation Wireless detection and monitoring is accomplished through a laptop-controlled Agilent E5071C network analyser connected to the 4 × 4 mm 2 readout printed antenna through a 12-inch SMA (SubMiniature version A) cable. The network analyser is controlled via USB VISA interface by a Matlab programme. Triggering of excitation and capturing of reflection spectrums, spectrum signal processing, resonance detection and graphical user interface output are all implemented in Matlab. For characterization measurements, input reflection spectra are averaged over 10 sweeps of 1,601 frequency points and white noise is removed with a 5-point medium filter. The same number of frequency points is captured without averaging and filtering in continuous monitoring studies. For pressure calibration curves, the same Matlab programme concurrently controls the chamber pressure by a Proportion Air QPV2 controller through National Instruments NI USB-6351 data acquisition device via a USB VISA interface. Gas pressure is supplied by a separate nitrogen gas tank. Wired pressure sensors are also read simultaneously to provide a pressure standard. In the saline studies, sensors are placed in a solution of 60 mM of NaCl in deionized water at room temperature. The depth of the solution is varied to characterize the separation range between the sensor and readout antenna. Pressure is applied by the N 2 gas pressure in the same chamber partially filled with saline. The sensor is placed at the bottom of the chamber in the fluid. This pressure is varied in the same manner as the air experiments, with the saline level kept fixed. For characterization of range in saline, sensors are allowed to float at the top of the variable-height water column and wirelessly detected through the bottom of the chamber. The depth of the solution is varied to characterize the separation range between the sensor and readout antenna. Pulse waveform monitoring A 2.5 × 2.5 mm 2 round sensor is placed on the radial artery of healthy adult subjects on the inside of the wrist and secured with silicone tape. Wireless monitoring is accomplished through a laptop-controlled Agilent E5071C network analyser connected to a 4 × 4 mm 2 readout printed antenna through a 12-inch SMA cable. The readout antenna is placed directly above the wireless surface sensor. The frequency sweep is adjusted to capture 501 points over a 200-MHz range for a pressure resolution below 0.5 mm Hg and a time resolution below 100 ms. In vivo validation All animal experiments were conducted according to the surgical protocol approved by the Administrative Panel on Laboratory Animal Care at Stanford University. Adult male C57BL/6 mice (30 g) were anaesthetized with 2.0% isoflurane and 1 l min −1 oxygen using a face mask, with the mice placed supine onto a stereotactic frame (Kopf Instruments, Tujunga, CA) and the head secured by ear bars. Using a dissection microscope, a 1-cm parasagittal incision was made to expose the coronal and superior sagittal sutures of the skull. An electric dental drill was used to create a small craniotomy window (4 × 5 mm 2 ) starting 2 mm lateral to the midline and 2 mm anterior to the coronal suture on the right side. The dura was opened and a 3 × 3 mm 2 sensor was slipped into the subdural space. The bone flap was replaced and secured using super glue. After the scalp incision was closed with sutures, an external 4 × 4 mm 2 readout antenna was placed directly adjacent to the implantation site. Wireless monitoring was accomplished through a laptop-controlled Agilent E5071C network analyser connected to the readout antenna through a 12-inch SMA cable. Pressure mapping Arrays of four 2 × 2 mm 2 sensor devices are designed in HFSS and co-simulated in Agilent Advanced Design System. The full array is fabricated by low-cost wax printing of each spiral layer on a shared substrate. Wireless monitoring is accomplished through a laptop-controlled Agilent E5071C network analyser connected to a single 4 × 4 mm 2 readout printed antenna through a 12-inch SMA cable. The readout antenna is placed directly above the centre point of the array. Uniform pressure is applied on the sensor inside a N 2 gas chamber whose pressure is regulated by a Proportion Air QPV2 controller through National Instruments NI USB-6351 data acquisition device via a USB VISA interface. Differential pressure is applied by gently pressing on the sensor s2 with the tip of a plastic tweezer. How to cite this article: Chen, L. Y. et al . Continuous wireless pressure monitoring and mapping with ultra-small passive sensors for health monitoring and critical care. Nat. Commun. 5:5028 doi: 10.1038/ncomms6028 (2014).